Controlling selectivities in CO2reduction through mechanistic understanding Catalytic CO 2 conversion to energy carriers and intermediates is of utmost importance to energy and environmental goals. However, the lack of fundamental understanding of the reaction mechanism renders designing a selective catalyst inefficient. Here we show the correlation between the kinetics of product formation and those of surface species conversion during CO 2 reduction over Pd/Al 2 O 3 catalysts. The operando transmission FTIR/SSITKA (Fourier transform infrared spectroscopy/steady-state isotopic transient kinetic analysis) experiments demonstrates that the rate-determining step for CO formation is the conversion of adsorbed formate, whereas that for CH 4 formation is the hydrogenation of adsorbed carbonyl. The balance of the hydrogenation kinetics between adsorbed formates and carbonyls governs the selectivities to CH 4 and CO. We apply this knowledge to the catalyst design and achieve high selectivities to desired products. Heterogeneous catalytic CO 2 reduction has been attracting great attention, because it not only mitigates the risks associated with increasing CO 2 concentration in the atmosphere but also offers a variety of pathways for producing fuels and industrial chemicals [1] , [2] . Under atmospheric pressure, methanation and reverse water gas shift (RWGS) reaction are the two pathways for thermocatalytic CO 2 reduction on Group VIII metals [2] . Although methanation produces synthetic natural gas, RWGS generates CO, an important component of syngas. Considerable efforts have been devoted to developing catalysts to achieve high selectivity towards either CH 4 or CO [3] , [4] , [5] , [6] , [7] , [8] , [9] . However, for designing a selective catalyst, it is very important to first have a fundamental understanding of the site requirements, elementary steps and intermediates, which can ultimately lead to the construction of viable mechanisms for both methanation and RWGS. Although intricate interplay between various surface species at different catalyst components that determine product selectivity has been recognized, controversies still exist regarding the detailed mechanism and the roles of surface species [10] , [11] , [12] , [13] , [14] , [15] . Some issues may originate from the different interrogation methods used; for example, some prior conclusions were based on kinetic and spectroscopic information acquired under transient conditions [12] . Under transient conditions, the perturbation of the chemical environment around the adsorbates and catalyst surface causes characteristically divergent behaviors from steady state. Steady-state isotopic transient kinetic analysis (SSITKA) has evolved as one of the most powerful techniques allowing measurements at steady state to determine the mean surface lifetimes and abundances of intermediates leading to products [16] , [17] . However, SSITKA itself cannot identify the chemical nature of surface species, a task that can be accomplished by operando spectroscopic measurements, e.g., Fourier transform infrared spectroscopy (FTIR). Correlating the reaction kinetics with the transformations of spectroscopically observable surface species, both simultaneously measured under steady-state reaction conditions, is vital for the complete elucidation of the complex mechanistic framework [18] , [19] , [20] , [21] . Pd-based catalysts are able to catalyze both CO 2 methanation and RWGS [22] , [23] . Our previous work on Pd/Al 2 O 3 bifunctional catalysts has proposed the plausible pathways for both CO 2 methanation and RWGS [24] . However, the factors that govern product selectivity (to CH 4 /CO) under steady-state CO 2 reduction conditions are still not clear. Here we show that CH 4 and CO selectivities are governed by the balance of the hydrogenation kinetics between adsorbed formates and carbonyls over Pd/Al 2 O 3 catalysts, which was demonstrated by a combined operando transmission FTIR spectroscopy/SSITKA investigation. Using this knowledge, we show that tailor-made catalysts can be prepared to achieve high selectivity to either of the two desired products. 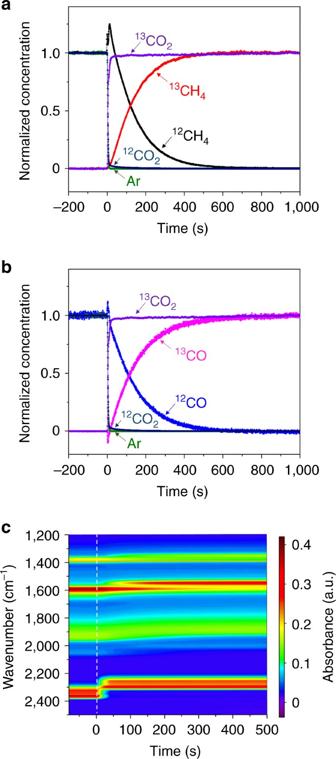Fig. 1 The responses of reactants, products and surface intermediates after the steady-state isotopic switch.a,bNormalized mass spectrometry signals of gases in the effluent andcFTIR contour plot collected as a function of time. The feed gas was switched at 0 s from12CO2/H2/Ar to13CO2/H2over 5% Pd/Al2O3at 533 K. Ar gas was used as an inert tracer Steady-state isotopic transient kinetic analysis Figure 1a, b show normalized mass spectrometry (MS) responses of gases in the effluent after the feed gas was switched at 0 s from 12 CO 2 /H 2 /Ar to 13 CO 2 /H 2 at 533 K. The fast disappearance of Ar gas in <4 s indicates a short gas hold-up time for the system. The disappearance of 12 CO 2 was almost as fast as Ar, indicating weak interaction between 12 CO 2 and the catalyst and the reactor walls. In the meantime, the concentration of 13 CO 2 signal increased accordingly, with the concentration and the conversion (2.5%) of carbon dioxide ( 12 CO 2 + 13 CO 2 ) constant during the switch. The decaying signals of 12 CH 4 and 12 CO and the rising signals of 13 CH 4 and 13 CO crossed at y = 0.5, indicating constant rates for methane and carbon monoxide formation regardless of isotopic substitution. These symmetrical responses indicate that the steady state of the catalyst surface was not perturbed during the switch. The concentrations of products 12 CH 4 and 12 CO decreased more slowly than that of 12 CO 2 and disappeared at ~600 s. This indicates large mean residence times for C-containing surface intermediates leading to the products, and that intermediates which equilibrate with CO 2 are not involved in the rate-determining steps for CO 2 methanation and RWGS. Fig. 1 The responses of reactants, products and surface intermediates after the steady-state isotopic switch. a , b Normalized mass spectrometry signals of gases in the effluent and c FTIR contour plot collected as a function of time. The feed gas was switched at 0 s from 12 CO 2 /H 2 /Ar to 13 CO 2 /H 2 over 5% Pd/Al 2 O 3 at 533 K. Ar gas was used as an inert tracer Full size image Figure 1c shows the corresponding operando FTIR contour plot. Before the switch, the absorption band between 2,300 and 2,400 cm −1 (red range) is attributed to gaseous 12 CO 2 . The spectral range between 1,800 and 2,100 cm −1 (blue and green range) is assigned to chemisorbed carbonyls ( ∗ 12 CO) on the surface of Pd metal particles [22] . The absorption bands around 1,400 (yellow range) and 1,600 cm −1 (red range) arise from adsorbed formates (H 12 COO ∗ ) on the surface of the Al 2 O 3 support [22] . After the switch, the bands due to 12 CO 2 quickly disappeared and a new band developed at lower wavenumbers (red range between 2,200 and 2,300 cm −1 ) attributable to 13 CO 2 , consistent with their rapid responses in MS. The IR signal decay of surface species might be slightly affected by the location of IR beam on the sample wafer [25] . However, the shift of the IR features of 12 CO ∗ and H 12 COO ∗ to those of 13 CO ∗ and H 13 COO ∗ at lower wavenumbers were much slower compared with the shift of 12 CO 2 to 13 CO 2 bands. This observation suggests that neither H 12 COO ∗ nor 12 CO ∗ undergoes reverse reactions to form 12 CO 2 . The disappearance trends of the IR signatures of H 12 COO ∗ and 12 CO ∗ are similar to those of the MS signals of 12 CH 4 and 12 CO products, suggesting that both H 12 COO ∗ and 12 CO ∗ are reactive intermediates rather than spectators and, the rate-determining steps for CH 4 and CO formation are related to CO ∗ and HCOO ∗ . It is noteworthy that no other species (e.g., bicarbonate) were observed under steady-state reaction conditions and no carbon deposition was identified in our previous study on Pd/Al 2 O 3 during CO 2 reduction [24] . Therefore, CO ∗ and HCOO ∗ are the two most abundant surface species and will be the focus of the following discussion. To gain insight into the interaction between ∗ CO and Pd on the 5% Pd/Al 2 O 3 , room temperature 12 CO adsorption followed by temperature-programed ∗ 12 CO desorption were studied by FTIR (Supplementary Fig. 1 ). At room temperature ∗ 12 CO on Pd showed IR features at 2,098, 2,052, 1,960 and 1,928 cm −1 . When the temperature was raised to 533 K, ∗ 12 CO with features at 2,098 and 1,960 cm −1 desorbed, whereas ∗ 12 CO with bands at 2,052 and 1,928 cm −1 did not desorb but was hydrogenated to CH 4 once H 2 was introduced. This reveals the existence of two types of adsorption sites on the Pd particles that bind CO weakly ( ∗ 12 CO w ) and strongly ( ∗ 12 CO s ). The stability of ∗ CO s at high temperatures is due to the dissociated ∗ H, which adsorbs near to ∗ CO s on the Pd surface and transfers electron density to Pd to strengthen the Pd-CO bond [22] , [26] . The FTIR spectrum of ∗ 12 CO s is very similar to that of ∗ 12 CO obtained in CO 2 reduction at 533 K, indicating that all ∗ 12 CO observed under reaction conditions were ∗ 12 CO s . However, ∗ 12 CO w could not be observed during CO 2 reduction at ≥ 533 K due to its rapid desorption. As we observe no ∗ 12 CO w under steady-state reaction conditions, the 12 CO product generated after the switch was mainly from the conversion of the other abundant species, H 12 COO ∗ . Normalized MS responses of 12 CH 4 and 12 CO with increasing temperature are shown in Supplementary Fig. 2 , whereas those for 13 CH 4 and 13 CO are not displayed. The faster decay in both 12 CH 4 and 12 CO signals at higher temperatures indicates the higher reactivities of intermediates. In contrast, the decay curves of 12 CO 2 and Ar did not change with temperature, further indicating that any elementary step that directly involves CO 2 is not the rate-limiting step for the formation of CH 4 and CO. The real mean surface residence times \({{{\bar \tau }}_{{0}}}\) (Supplementary Fig. 3 ) of intermediates leading to 12 CH 4 and 12 CO (denoted as ICH and ICO) together with the \({{{\bar \tau }}_{{0}}}\) -derived activation energies E for 12 CH 4 and 12 CO formation (Supplementary Fig. 4 ) are summarized in Table 1 . The \({{{ \bar \tau }}_{{{0}}\_{{\rm ICH}}}}\) at 533 K was 134 s and gradually decreases with increasing temperature, reaching 41 s at 573 K. Similarly, the \({{{ \bar \tau }}_{{{0}}\_{{\rm ICO}}}}\) decreased from 107 to 55 s with increasing temperature from 533 to 573 K. The activation energies are 75 and 53 kJ mol −1 for the formation of CH 4 and CO, respectively, in line with the values we obtained previously in a plug-flow reactor [24] . Series of corresponding operando FTIR spectra of ∗ CO and HCOO ∗ collected at 533–573 K are shown in Supplementary Figs. 5 , 6 , respectively. The shift of IR bands representing ∗ 12 CO s and H 12 COO ∗ to those representing ∗ 13 CO s and H 13 COO ∗ became faster with increasing temperature, but still remained much slower than the shift of the IR band of 12 CO 2 to that of 13 CO 2 . The decay trends of ∗ 12 CO s and H 12 COO ∗ FTIR intensity with increasing temperature was very similar to the decay trends of MS signals of 12 CH 4 and 12 CO products (Supplementary Fig. 2 ), further indicating that HCOO ∗ and CO ∗ are related to the rate determining steps for CO and CH 4 formation. In addition, the disappearances of ∗ 12 CO s and H 12 COO ∗ follow an apparent first-order kinetics. The activation energies based on the Arrhenius plots of the two first-order rate constants (Supplementary Figs. 5 , 6 ) are listed in Table 1 . The activation energy for the conversion of ∗ 12 CO s was 73 kJ mol −1 , an identical value to that determined for 12 CH 4 formation from the MS data. This result suggests that the rate-determining step along the CH 4 formation path is the conversion of ∗ CO s . The activation energy of H 12 COO ∗ conversion was 52 kJ mol −1 , very similar to the 53 kJ mol −1 determined for the 12 CO formation by MS, indicating that the conversion of HCOO ∗ is the rate-determining step for CO formation. 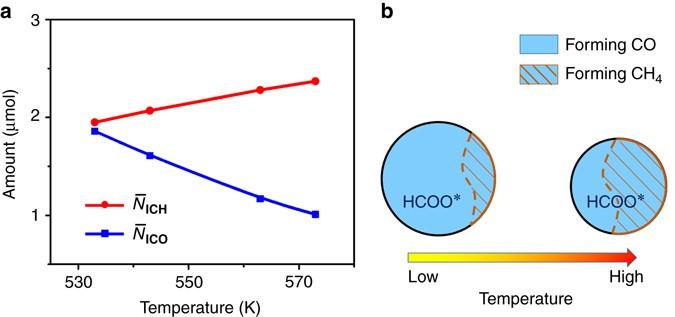Fig. 2 The distribution of surface intermediates in the pathways under steady state.aThe amount of surface intermediates leading to12CH4\(\left( {{{{{\bar N}}}_{{{\rm ICH}}}}} \right)\)and12CO\(\left( {{{{{ \bar N}}}_{{{\rm ICO}}}}} \right)\)on the catalyst (41 mg) during CO2reduction at 533–573 K.bSchematic representation of the proportion of surface coverage of HCOO∗that is eventually converted to CH4and CO with increasing temperature concluded froma Table 1 Real mean surface residence times for ICH \(\left( {{{{{ \bar \tau }}}_{{{0}}\_{{\rm ICH}}}}} \right)\) and ICO \(\left( {{{{{ \bar \tau }}}_{{{0}}\_{{\rm ICO}}}}} \right)\) , and activation energies for CH 4 ( E CH4 ) and CO ( E CO ) formation and adsorbed ∗ COs ( E ∗ COs) and HCOO ∗ ( E HCOO ∗ ) conversions in CO 2 reduction at 533–573 K Full size table Abundance of surface intermediates Figure 2 shows the surface abundance \(\left( {{{ \bar N}}} \right)\) of ICH and ICO from SSITKA at 533–573 K. The \({{{ \bar N}}_{{{\rm ICO}}}}\) was 1.86 μmol at 533 K, and decreased to 1.01 μmol as the temperature was increased to 573 K. As demonstrated above, 12 CO was produced from the existing H 12 COO ∗ . Thus, the amount of H 12 COO ∗ that was converted to 12 CO was less at higher temperatures than at lower temperatures. In contrast, the \({{{ \bar N}}_{{{\rm ICH}}}}\) increased from 1.95 μmol at 533 K to 2.37 μmol at 573 K. This increase could be interpreted as being caused by an increased concentration of ∗ 12 CO s at higher temperatures. However, this is not the case, as no difference in intensity of ∗ 12 CO s was observed as the temperature was increased from 533 to 573 K (Supplementary Fig. 7 ). The constant intensity of ∗ 12 CO s implies that the amount of 12 CH 4 produced from ∗ 12 CO s , which have already existed at the moment of the switch, should be the same at 533–573 K. Therefore, the significant increase in the amount of 12 CH 4 at higher temperatures is attributed to the conversion of the other abundant species, H 12 COO ∗ . These results suggest that with increasing temperature, for a given amount of surface HCOO ∗ at steady state, a progressively larger portion enters the CO 2 methanation pathway, while a smaller portion enters the RWGS pathway (Fig. 2b ). This explains the decreased \({{{ \bar N}}_{{{\rm ICO}}}}\) at higher temperature. This also agrees well with the above SSITKA results, which show that the \({{{ \bar \tau }}_{{{0}}\_{{\rm ICH}}}}\) became shorter than \({{{ \bar \tau }}_{{{0}}\_{{\rm ICO}}}}\) with increasing temperature. Therefore, formates prefer to enter the faster pathway to form CH 4 rather than enter the slower pathway to form CO at higher temperature. Similarly, Goodwin et al. discussed a case where two products share an intermediate: if \({{{ \bar \tau }}_{{1}}}\) > \({{{ \bar \tau }}_{{2}}}\) , then it must be that \({{{ \bar N}}_{{1}}}\) < \({{{ \bar N}}_{{2}}}\) , because more of this intermediate will form product 2 than product 1 due to the faster formation of product 2 (smaller \({{{ \bar \tau }}_{{2}}}\) ) [27] . Therefore, the temperature effect on these parameters, \({{{ \bar \tau }}_{{{0}}\_{{\rm ICH}}}}\) , \({{{ \bar \tau }}_{{{0}}\_{{\rm ICO}}}}\) , \({{{ \bar N}}_{{{\rm ICH}}}}\) and \({{{\bar N}}_{{{\rm ICO}}}}\) , further demonstrates that HCOO ∗ is the intermediate shared by the processes of both CO 2 methanation and RWGS. Fig. 2 The distribution of surface intermediates in the pathways under steady state. a The amount of surface intermediates leading to 12 CH 4 \(\left( {{{{{\bar N}}}_{{{\rm ICH}}}}} \right)\) and 12 CO \(\left( {{{{{ \bar N}}}_{{{\rm ICO}}}}} \right)\) on the catalyst (41 mg) during CO 2 reduction at 533–573 K. b Schematic representation of the proportion of surface coverage of HCOO ∗ that is eventually converted to CH 4 and CO with increasing temperature concluded from a Full size image Based on above results and SSITKA theory [16] , [17] , a scheme relating HCOO ∗ , ∗ CO s and ∗ CO w species in CO 2 reduction is proposed in Fig. 3 . The reduction of formate produces ∗ CO that first occupies strong adsorption sites on the Pd particles. Once the strong adsorption sites of Pd particles are saturated (the pool of ∗ CO s is completely filled), the excess ∗ CO can only occupy the weak adsorption sites of Pd particles to form ∗ CO w . The ∗ CO s will be further hydrogenated to CH 4 while the ∗ CO w will desorb. Fig. 3 Factors governing the selectivities in CO 2 reduction. Scheme for the pathways from formate to products in CO 2 methanation and RWGS over Pd/Al 2 O 3 catalysts. The filled pool of ∗ CO s and the unfilled pool of HCOO ∗ are supported by the unchanged coverage of ∗ 12 CO s and the changed coverage of H 12 COO ∗ at 533–573 K (Supplementary Fig. 7 ) Full size image The scheme shows that the rate of CO formation ( r CO ) is determined and equal to the rate of HCOO ∗ conversion ( \({r_{{\rm{HCOO}}^{*}}}\) ) subtracted by the rate of CH 4 formation ( r CH4 ): 
    r_CO = r_HCOO^* - r_CH4
 (1) The rate of CH 4 formation is equal to the rate of ∗ CO s conversion ( \({r_{{\,}^{*}{\rm{COs}}}}\) , the rate-determining step for CH 4 formation), which is proportional to the concentration of ∗ CO s . The completely filled pool of ∗ CO s in the 533–573 K temperature range suggests that \({r_{{\,}^{*}{\rm{COs}}}}\) has reached its maximum, \({r_{{\,}^{*}{\rm{COs}}\_{\rm{max}}}}\) , at each given temperature between 533–573 K. Therefore, it is the balance between the rate of HCOO ∗ reduction to ∗ CO ( \({r_{{\rm{HCOO}}^{*}}}\) ) and the maximum rate of ∗ CO s conversion ( \({r_{{\,}^{*}{\rm{COs}}\_{\rm{max}}}}\) ) that determines whether CO is observed in the gas phase or not. If \({r_{{\rm{HCOO}}^{*}}}\) > \({r_{{\,}^{*}{\rm{COs}}\_{\rm{max}}}}\) , both CH 4 and CO will be observed (e.g., the case in Fig. 3 ). If, however, \({r_{{\rm{HCOO}}^{*}}}\) ≤ \({r_{{\,}^{*}{\rm{COs}}\_{\rm{max}}}}\) , which means that all the ∗ CO produced from HCOO ∗ are not sufficient to saturate all strong adsorption sites on the Pd metal for CH 4 formation (i.e., the pool of ∗ CO s in Fig. 3 is not full or just full), then all ∗ CO will be ∗ CO s and will be further hydrogenated to CH 4 . In this case, CO 2 reduction will only be methanation and the rate of CH 4 formation r CH4 ( \({r_{{\,}^{*}{\rm{COs}}}}\) ) will not reach its maximum \({r_{{\,}^{*}{\rm{COs}}\_{\rm{max}}}}\) . As the conversions of both HCOO ∗ and ∗ CO s require the presence of ∗ H (absorbed hydrogen) involved [24] , r CH4 ( \({r_{{\,}^{*}{\rm{COs}}\_{\rm{max}}}}\) ) is determined by the concentrations of ∗ CO s ([ ∗ CO s ]) and ∗ H ([ ∗ H]), as well as the rate constant of ∗ CO s conversion ( k 1 ): 
    r_CH4 = r*_COs_max = k_1[  ^*CO_s][  ^*H]
 (2) and \({r_{{\rm{HCOO}}^{*}}}\) is determined by the concentration of HCOO ∗ ([HCOO ∗ ]) and ∗ H ([ ∗ H]), and rate constant of HCOO ∗ reduction ( k 2 ): 
    r_HCOO* = k_2[ HCOO^*][ ^*H],
 (3) so 
    r_CO = r_HCOO* - r_CH4 = r_HCOO* - r*_COs_max
     = k_2[ HCOO^*][  ^* H] - k_1[ ^* CO_s][  ^* H]1.2pc
 (4) It is known that ∗ CO s and HCOO ∗ do not share and compete for active sites, as they are located on Pd metal and Al 2 O 3 support, respectively [22] . Therefore, [ ∗ CO s ] and [HCOO ∗ ] can be independently changed to tune the rate of CO formation, r CO , as well as the reaction product distribution. In the case of a completely filled pool of ∗ CO s (e.g., the case in Fig. 3 ), if aiming at a higher CH 4 selectivity, [ ∗ CO s ] should be increased or [HCOO ∗ ] should be decreased. One method, e.g., is to add more metal sites onto the Al 2 O 3 support. The increased metal loading will not only result in an increased number of metal sites for forming ∗ CO s but also lead to a decreased number of support sites that can accommodate HCOO ∗ . It means that the capacity of ∗ CO s pool (Fig. 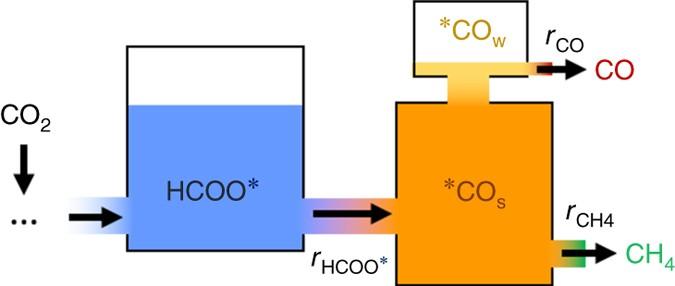Fig. 3 Factors governing the selectivities in CO2reduction. Scheme for the pathways from formate to products in CO2methanation and RWGS over Pd/Al2O3catalysts. The filled pool of∗COsand the unfilled pool of HCOO∗are supported by the unchanged coverage of∗12COsand the changed coverage of H12COO∗at 533–573 K (Supplementary Fig.7) 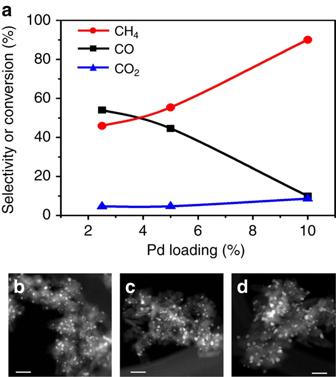Fig. 4 Controlled selectivities in CO2reduction by tailor-made catalysts through mechanistic understanding.aCH4and CO selectivities and CO2conversion as a function of Pd loading at 573 K.b–dSTEM images of 2.5, 5 and 10% Pd/Al2O3. STEM scale bars represent 20 nm. (Particle size distributions and temperature-programed∗12CO desorption for the catalysts are displayed in Supplementary Fig.8) 3 ) is enlarged, meanwhile that of HCOO ∗ is decreased. This, consequently, may lead to a situation where the result of Eq. ( 4 ) decreases even to 0, showing less or complete absence of CO in the gas phase. This hypothesis was tested on Pd/Al 2 O 3 catalysts with different Pd loadings but similar Pd particle size distributions (Fig. 4 ), which minimized the potential effects of metal particle size on k 1 and k 2 influencing \({r_{{\,}^{*}{\rm{COs}}\_{\rm{max}}}}\) and \({r_{{\rm{HCOO}}^{*}}}\) . If the scheme and hypothesis are correct, Pd/Al 2 O 3 catalysts with higher Pd loadings should exhibit higher CH 4 selectivity than those with lower Pd loadings. Furthermore, this is exactly what the reactivity data of Fig. 4 shows: CH 4 selectivity increased from 45 to 90% as the Pd loading was increased from 2.5 to 10% (Fig. 4 ). Previous studies on Ru/Al 2 O 3 and Ni/SiO 2 catalysts have also shown that CH 4 selectivity in CO 2 reduction reaction increased with the metal loading [12] , [28] , [29] , consistent with the findings reported in this work. Fig. 4 Controlled selectivities in CO 2 reduction by tailor-made catalysts through mechanistic understanding. a CH 4 and CO selectivities and CO 2 conversion as a function of Pd loading at 573 K. b – d STEM images of 2.5, 5 and 10% Pd/Al 2 O 3 . STEM scale bars represent 20 nm. (Particle size distributions and temperature-programed ∗ 12 CO desorption for the catalysts are displayed in Supplementary Fig. 8 ) Full size image In the case of an incompletely filled pool of ∗ CO s, when CH 4 selectivity is always 100%, if one aims at a higher CH 4 formation rate, [ ∗ CO s ] needs to be increased. For instance, Karelovic et al. [30] reported that the rate of CO 2 methanation over Rh/Al 2 O 3 was greatly increased by adding Pd/Al 2 O 3 , which has no activity towards CO 2 methanation at 473 K. They attributed the synergistic effect to the supply of dissociated H ∗ from Rh/Al 2 O 3 to Pd/Al 2 O 3 . It is noteworthy that although CO 2 methanation cannot proceed on Pd/Al 2 O 3 at 473 K, this temperature is high enough for RWGS reaction to occur producing CO [22] , [31] . We propose that CO or ∗ CO produced by/on Pd/Al 2 O 3 could diffuse onto the Rh domains, increasing the concentration of ∗ CO s on Rh. The total amount of ∗ CO s produced by both Pd/Al 2 O 3 and Rh/Al 2 O 3 is still not enough to saturate all the active Rh sites for CH 4 formation (to fill up the ∗ CO s pool of Rh, Fig. 3 ). Therefore, the CH 4 selectivity remained ~100% but the methanation rate was higher on the Pd/Al 2 O 3 -Rh/Al 2 O 3 mixture than on Rh/Al 2 O 3 alone. The role of the Pd/Al 2 O 3 component was to provide extra CO ( ∗ CO) to the empty sites of Rh. The synergistic effect at lower catalyst temperature (423 K) was found to be negligible. Our study showed that RWGS cannot occur over Pd/Al 2 O 3 at 423 K [31] , so the added Pd/Al 2 O 3 cannot supply additional CO to Rh/Al 2 O 3 catalyst for the further ∗ CO hydrogenation to CH 4 on Rh/Al 2 O 3 . Therefore, the above analysis of their results show that for an incompletely filled pool of ∗ CO s with 100% CH 4 selectivity ( \({r_{{\rm{HCOO}}^{*}}}\) ≤ \({r_{{\,}^{*}{\rm{COs}}\_{\rm{max}}}}\) ) on a catalyst, adding a component (promoter) which can produce CO ( ∗ CO) is a strategy for increasing the rate of CO 2 methanation. In conclusion, CO 2 methanation and RWGS are not two parallel reactions during the CO 2 reduction over Pd/Al 2 O 3 catalysts. Instead, they share the initial steps and intermediates from bicarbonates to formates until after formate decomposition. The rate of formate decomposition to CO ∗ is larger than the rate of ∗ CO hydrogenation to CH 4 and the excess CO ∗ desorbs. The rate-determining step for CO 2 reduction and for RWGS is the conversion of HCOO ∗ , whereas that for CH 4 formation is the hydrogenation of ∗ CO. The balance of the hydrogenation kinetics between HCOO ∗ and ∗ CO governs the selectivities to CH 4 and CO. Given that ∗ CO and HCOO ∗ are mainly on metal (Pd) and support (Al 2 O 3 ), respectively, the balance could be tuned to achieve the desired CH 4 and CO selectivities by optimizing the loading of the metal and the surface area of the support. This work has important implications for other bifunctional systems where the balance between different catalytic functions determines the rates and product distribution. Catalyst synthesis and SSITKA experiments The Pd/Al 2 O 3 catalysts were prepared on a γ-Al 2 O 3 powder (Sasol, Puralox SBA-200) by the incipient wetness method using Pd(NH 3 ) 4 (NO 3 ) 2 as the precursor. After impregnation, the samples were dried at 373 K for 24 h and then calcined at 773 K for 2 h in air (flow rate = 60 mL min −1 ) and followed by reduction at 773 K for 1 h in 10% H 2 /He (flow rate = 60 mL min −1 ) to obtain the Pd/Al 2 O 3 catalysts [31] . Forty-one milligrams of 5 wt% Pd/Al 2 O 3 was pressed onto a tungsten mesh and loaded into a home-made operando transmission IR cell [32] . The cell has a very small internal dead volume (~0.2 cm 3 after the catalyst loading), resulting in a short gas hold-up time. This renders the system suitable for obtaining accurate kinetic information about intermediates and products during the SSITKA experiments. Before experiments, the catalyst was pretreated by calcination at 673 K for 1 h under air with a flow rate of 10 mL min −1 , followed by reduction at 673 K for 1 h under 20% H 2 in He with a flow rate of 10 mL min −1 . The reactant gas mixture was composed of 4 mL min −1 H 2 , 1 mL min −1 12 CO 2 or 13 CO 2 , 1 mL min −1 Ar and He as the diluent with a total gas flow of 10 mL min −1 at atmospheric pressure. Ar gas was used as an inert tracer to correct for gas hold-up of the system and for gas re-adsorption. After the reaction reached steady state at the reaction temperature of 533 K, the reactant was switched from H 2 / 12 CO 2 /Ar to H 2 / 13 CO 2 . During the switch, the gaseous effluent from the cell and the species on the catalyst surface were monitored by MS and FTIR, respectively. The switch was performed in the temperature range of 533–573 K, where the CO 2 conversion was <8%. In order to obtain the real mean surface residence times ( \({{{ \bar \tau }}_{{0}}}\) ) of intermediates leading to CH 4 and CO, space velocity experiments were conducted by varying the total flow rate from 10 to 25 mL min −1 at constant partial pressures of CO 2 and H 2 to exclude gas hold-up and re-adsorption effects. Data analysis The SSITKA theory has earlier been described extensively [16] , [33] . The integration of the normalized step-decay or step-input response always yields the overall mean surface-residence time, \({{ \bar \tau }}\) , of all adsorbed surface intermediates, which lead to CH 4 and CO products \(\left( {{{ \bar \tau }} = {\int}_0^\infty {F(t){\rm{d}}t} } \right)\) . The error <5% caused by gas phase hold-up (~3 s) could be ignored due to the fast decay of standard Ar gas and CO 2 gas. The rate constant is simply the reciprocal of average surface residence time for the active surface intermediates ( k = \({{{ \bar \tau }}^{ - {\rm{1}}}}\) = TOF ∗ θ −1 ). The number of adsorbed species \(\left( {{{{{ \bar N}}}_{{{\rm ICH}}}}} \right)\) and CO \(\left( {{{{{ \bar N}}}_{{{\rm ICO}}}}} \right)\) can be obtained from integration of decay rates ( r ) of CH 4 and CO products \(\left( {\bar N = {\int}_0^\infty {r(t){\rm{d}}t} } \right)\) . In addition, \({{ \bar N}}\) is usually closely related to the number of active sites on the catalysts for product formation. In this study of CO 2 reduction over 41 mg of 5% Pd/Al 2 O 3 , the \({{{ \bar N}}_{{{\rm ICO}}}}\) completely originates from H 12 COO ∗ , which was demonstrated to be located on the Al 2 O 3 support. As not all H 12 COO ∗ was converted to 12 CO, the amount of sites for formates on Al 2 O 3 is estimated to be at least 1.86 μmol, i.e., \({{{ \bar N}}_{{{\rm ICO}}}}\) obtained at 533 K. For CH 4 formation via ∗ 12 CO s and a portion of H 12 COO ∗ , the upper limit of the amount of active Pd sites for ∗ CO s (forming CH 4 ) is 1.95 μmol, i.e., \({{{ \bar N}}_{{{\rm ICH}}}}\) at 533 K. This value accounts for 90% of the surface Pd atoms. The total amount of intermediates ( \({{{ \bar N}}_{{{\rm CO}}}}\) + \({{{ \bar N}}_{{{\rm CH4}}}}\) ) on the surface of the catalyst slightly decreased from 3.81 μmol at 533 K to 3.38 μmol at 573 K, which was caused by the decreased amount of H 12 COO ∗ on the surface shown in Supplementary Fig. 7 . Data availability The data that support the findings of this study are available from the corresponding author on request.